Malaria parasite tyrosyl-tRNA synthetase secretion triggers pro-inflammatory responses Malaria infection triggers pro-inflammatory responses in humans that are detrimental to host health. Parasite-induced enhancement in cytokine levels correlate with malaria-associated pathologies. Here we show that parasite tyrosyl-tRNA synthetase ( Pf TyrRS), a housekeeping protein translation enzyme, induces pro-inflammatory responses from host immune cells. Pf TyrRS exits from the parasite cytoplasm into the infected red blood cell (iRBC) cytoplasm, from where it is released into the extracellular medium on iRBC lysis. Using its ELR peptide motif, Pf TyrRS specifically binds to and internalizes into host macrophages, leading to enhanced secretion of the pro-inflammatory cytokines TNF-α and IL-6. Pf TyrRS-macrophage interaction also augments expression of adherence-linked host endothelial receptors ICAM-1 and VCAM-1. Our description of Pf TyrRS as a parasite-secreted protein that triggers pro-inflammatory host responses, along with its atomic resolution crystal structure in complex with tyrosyl-adenylate, provides a novel platform for targeting Pf TyrRS in anti-parasitic strategies. Aminoacyl-tRNA synthetases are ancient enzymes responsible for genetic code translation [1] . These ubiquitous enzymes attach amino acids onto cognate transfer RNAs during protein translation, and are divided into two classes based on their structural topology [1] , [2] . Class I synthetases, like tyrosyl-tRNA synthetase (TyrRS), are characterized by a Rossmann fold, and this class contains two conserved ATP-binding motifs (HIGH and KMSKS) [3] , [4] . Apart from their parent aminoacylation activity, several aminoacyl-tRNA synthetases perform non-canonical functions in transcriptional regulation, apoptosis, ribosomal RNA biogenesis, angiogenesis and cell signalling [5] , [6] , [7] , [8] . Human TyrRS is processed by an elastase enzyme yielding an amino-terminal TyrRS (also known as mini-TyrRS) and carboxy-terminal EMAPII-like domain [9] , [10] , [11] , [12] , [13] . The latter contains cell signalling activity whereas human mini-TyrRS mimics interleukin-8 (IL-8) to chemo-attract polymorphonuclear cells [9] , [10] , [11] , [12] , [13] . Human mini-TyrRS interacts with CXCR1/2 receptors and acts as an angiogenic cytokine using a motif called ELR (Glu-Leu-Arg) that it shares with IL-8 ( Fig. 1a ). For the human mini-TyrRS ELR motif to be functional, the intact human enzyme is required to undergo proteolytic cleavage, which results in the release of EMAPII domain and subsequent exposure of the ELR motif [9] , [10] , [11] , [12] , [13] . 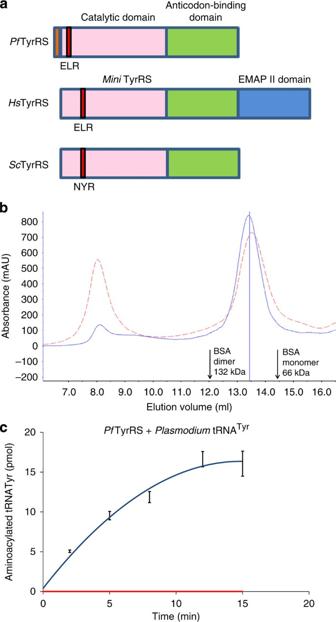Figure 1: Tyrosyl tRNA synthetase domain organization and enzyme characterization. (a) Domain organization of TyrRS fromP. falciparum, human and yeast. The 21 residue N-terminal extension inPfTyrRS is shown in orange. The ELR motif is shown in red and in yeast TyrRS it is replaced by NYR. (b) Gel filtration curves show both wild-typePfTyrRS (solid blue line) and ELR/AAA mutant (dotted red line) proteins as dimers in solution. (c) Aminoacylation curves with (blue line) and without (red line) added nativePfTyrRS and usingPf-tRNATyr. Figure 1: Tyrosyl tRNA synthetase domain organization and enzyme characterization. ( a ) Domain organization of TyrRS from P. falciparum , human and yeast. The 21 residue N-terminal extension in Pf TyrRS is shown in orange. The ELR motif is shown in red and in yeast TyrRS it is replaced by NYR. ( b ) Gel filtration curves show both wild-type Pf TyrRS (solid blue line) and ELR/AAA mutant (dotted red line) proteins as dimers in solution. ( c ) Aminoacylation curves with (blue line) and without (red line) added native Pf TyrRS and using Pf -tRNA Tyr . Full size image Plasmodium parasites are the causative agents of malaria. It is estimated that >300 million clinical malaria cases occur annually, resulting in >1 million deaths [14] . Malaria-related deaths occur owing to a range of syndromes including acute anemia and/or cerebral/placental malaria [14] , [15] . Most malaria pathology results from an acute inflammatory spurt, followed by activation of the host immune system and dysregulated cytokine release [14] , [15] , [16] , [17] , [18] . Human patient studies and mouse malaria models have consistently suggested that infection by the malaria parasite triggers an increase in the levels of numerous pro-inflammatory agents including tumour necrosis factor (TNF-α), interferon gamma (IFN-γ) and interleukin 6 (IL-6) in blood plasma [19] , [20] , [21] . Although pro-inflammatory cytokines have a major role in patho-physiology of malaria disease [16] , [17] , [18] , [19] , [20] , [21] , the molecular mechanisms of cytokine release from immune cells remains largely unclear. Until now, several parasite-derived molecular agents have been implicated in triggering cytokine release [22] , [23] , [24] , [25] , but parasite-secreted protein(s) that potentially trigger specific cytokine secretion from host immune cells are less well understood. It is critical to understand the pathways and mechanisms that lead to cytokine release in malaria as disease pathology, directly or indirectly, generally results from dysregulation of circulating TNF-α and IL-6 amounts [22] , [23] , [24] , [25] . Plasmodium falciparum genome contains two copies of tyrosyl-tRNA synthetase-tyrosyl-tRNA synthetase 1 (hereafter Pf TyrRS, Plasmodb ID=MAL8p1.125) and tyrosyl-tRNA synthetase 2 (hereafter Pf TyrRS api , Plasmodb ID=PF11_0181). Pf TyrRS was predicted to be cytoplasmic whereas Pf TyrRS api is probably targeted to the parasite apicoplast [6] . Here we have investigated the structural, immunological and spatial localization attributes of Pf TyrRS. Our comprehensive analyses provide a platform for focusing on Pf TyrRS as a new target for development of novel malaria intervention strategies. Pf TyrRS characterization and structure Bacterially overexpressed Pf TyrRS was purified to homogeneity using affinity and gel-filtration chromatography, and the protein migrates as a dimer ( Fig. 1b ). Pf TyrRS enzyme activity was confirmed using tRNAs obtained by in vitro transcription using T7 RNA polymerase ( Fig. 1c ) [26] , [27] , [28] . We determined the three-dimensional structure of Pf TyrRS in complex with YAP (tyrosyl-adenylate) to a resolution of 2.2 Å ( Fig. 2a,b; Table 1 ). The crystallographic asymmetric unit contains a canonical tyrosyl-tRNA synthetase dimer. Eighteen N-terminal and three C-terminal residues were not clearly defined in the electron density for each monomer. The overall fold of Pf TyrRS is typical of class I synthetases [3] , [4] and comprises a catalytic domain (residues 18–260, Rossmann fold) and an anti-codon-binding domain (residues 261–370). Human mitochondrial and malaria parasite apicoplastic TyrRS belong to bacterial lineage, whereas human cytoplasmic TyrRS and Pf TyrRS belong to a separate eukaryotic group [6] , [29] ( Fig. 2c ). Structural superposition of 292 C α atoms between Pf TyrRS and human mini-TyrRS (Protein Data Bank, accession code 1N3 L) gives an RMSD of ∼ 1.9 Å (sequence identity ∼ 30%), whereas the RMSD between 144 C α atoms of Pf TyrRS and mitochondrial Hs TyrRS (PDB: 2PID ) is ∼ 2.5 Å (sequence identity <10%). In Pf TyrRS, the solvent accessible buried surface area at dimer interface is ∼ 1,337 Å 2 , and its value is comparable with L -Tyr bound mini- Hs TyrRS (1,380 Å 2 ) but not with the unliganded mini- Hs TyrRS (buried area of 1,531 Å 2 ). In mini- Hs TyrRS structure [13] , the adenosine binding pocket is empty and seems enlarged by ∼ 3 Å on either side of the binding pocket whereas, in YSA (5′-O-[N-( L -Tyrosyl) sulfamoyl] adenosine)-bound mitochondrial Hs TyrRS [29] and in YAP-bound Pf TyrRS, the adenosine-binding pocket is tighter ( Fig. 2d ). In Pf TyrRS, the key synthetase motif of KMSKS loop is highly ordered and close to the bound substrate at the active site, whereas, in both cytoplasmic and mitochondrial Hs TyrRS, this is found to be disordered ( Fig. 2d ). We find several other key structural differences between mini- Hs TyrRS and Pf TyrRS ( Fig. 2c,d ). First, at the primary sequence level, Pf TyrRS has an N-terminal 21 residue extension whose role is unclear ( Fig. 1a ). On the other hand, human cytoplasmic TyrRS has a C-terminal extension in the form of an EMAPII domain that undergoes proteolytic processing to reveal a host module more similar in size to Pf TyrRS [9] , [10] , [11] , [12] , [13] ( Fig. 1a ). The most notable and intriguing feature of both the mini- Hs TyrRS and Pf TyrRS is presence of an ELR motif ( Figs. 1a and 2e ). This tri-peptide signature is present in, among others, cytokines like IL-8 (refs 9 , 10 , 11 , 12 , 13 , 30 ). 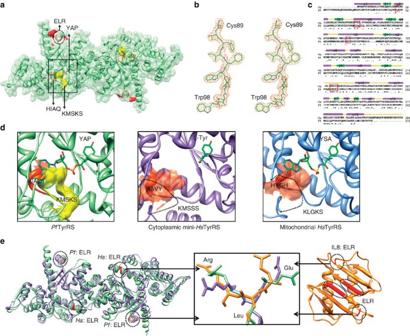Figure 2: Crystal structure ofPfTyrRS. (a)PfTyrRS:Tyr-AMP (YAP) complex structure where the ELR, KMSKS and HIGH motifs are shown in red, yellow and orange, respectively. Bound YAP is shown in stick model (green). (b) Stereoview of the experimental electron density map (2|Fo|-|Fc|) for a portion of the final atomic model. The map is contoured at 1.2 σ level. (c) Sequence alignment between mini-HsTyrRS andPfTyrRS. Important motifs are highlighted in red boxes and the ELR motifs are marked. (d) A close-up view of KMSKS loop and active site region ofPfTyrRS along with corresponding regions from cytoplasmic mini-HsTyrRS and mitochondrialHsTyrRS (with 5′-O-[N-(L-Tyrosyl) sulfamoyl] adenosine also known as YSA). The disordered KMSKS loop is shown as dotted lines in human structures and the bound substrate/analog is shown as sticks. (e) Structural alignment and ELR motifs in mini-HsTyrRS (purple),PfTyrRS (green) andHsIL-8 (orange). As shown in Figure 2e , ELR motifs decorate the surfaces of IL-8, mini- Hs TyrRS and Pf TyrRS. Structural alignment of ELR motifs from these three reveals striking conformational conservation (RMSD <1 Å). In Pf TyrRS, the ELR motif resides on α-helix 2 whereas, in mini- Hs TyrRS, it is located at α-helix 5 ( Fig. 2e ). In both Pf TyrRS and mini- Hs TyrRS, the ELR motif is significantly distal from aminoacylation sites ( Fig. 2e ). In full-length cytoplasmic Hs TyrRS, the ELR motif is buried under the C-terminal EMAPII domain, and this motif is exposed after proteolytic cleavage [9] , [10] , [11] , [12] , [13] . In contrast, the Pf TyrRS ELR motif is exposed in three-dimensional space and does not require processing for its surface display. Therefore, in the parasite enzyme the ELR tri-peptide is continually solvent accessible owing to its presence in a different part of the overall three-dimensional structure relative to human TyrRS ( Fig. 2a,e ). Subtle structural perturbations caused by single residue mutations near the ELR motif can activate procytokine activity of human TyrRS [11] . These data on human TyrRS [11] suggested that the twin attributes of cytokine trigger and aminoacylation can coexist in a tyrosyl-tRNA synthetase [11] . Indeed, our description of the parasite Pf TyrRS provides an excellent natural example of a synthetase enzyme with constitutively active ELR motif ( Fig. 2 ). Interestingly, the ELR motif is absent in TyrRSs from lower eukaryotes and prokaryotes ( Fig. 1a ), again suggesting that ELR motif is independent of the parent aminoacylation activity of these enzymes. Figure 2: Crystal structure of Pf TyrRS. ( a ) Pf TyrRS:Tyr-AMP (YAP) complex structure where the ELR, KMSKS and HIGH motifs are shown in red, yellow and orange, respectively. Bound YAP is shown in stick model (green). ( b ) Stereoview of the experimental electron density map (2|Fo|-|Fc|) for a portion of the final atomic model. The map is contoured at 1.2 σ level. ( c ) Sequence alignment between mini -Hs TyrRS and Pf TyrRS. Important motifs are highlighted in red boxes and the ELR motifs are marked. ( d ) A close-up view of KMSKS loop and active site region of Pf TyrRS along with corresponding regions from cytoplasmic mini- Hs TyrRS and mitochondrial Hs TyrRS (with 5′-O-[N-( L -Tyrosyl) sulfamoyl] adenosine also known as YSA). The disordered KMSKS loop is shown as dotted lines in human structures and the bound substrate/analog is shown as sticks. ( e ) Structural alignment and ELR motifs in mini- Hs TyrRS (purple), Pf TyrRS (green) and Hs IL-8 (orange). Full size image Table 1 Data collection and refinement statistics. Full size table Structural comparisons suggest sequence differences in 11 key residues that contribute to L -Tyr binding (5 residues) and adenosine binding (6 residues) between human and parasite enzymes ( Fig. 2c,d ). Residues in the conserved HIGH and KMSKS motifs are different between Pf TyrRS (HIAQ and KMSKS) and mini- Hs TyrRS (HAVY and KMSSS). In the L -Tyr bound mini- Hs TyrRS, a K + ion is bound near adenine binding pocket whereas this space is empty in unliganded state of mini- Hs TyrRS. In Pf TyrRS, there is no density for an ion like K + , and further the residues involved in K + ion coordination in mini- Hs TyrRS are not conserved in Pf TyrRS. Therefore, several subtle yet crucial differences between host and pathogen tyrosyl-tRNA synthetase active sites ( Fig. 2b–d ) present a window for exploiting the malaria parasite enzyme for structure-based inhibitor discovery—consistent with recent high-throughput chemical library screening data [31] . Parasite and erythrocyte localization of Pf TyrRS Confocal microscopy was performed using protein-A purified IgG fraction of rabbit antibodies that were raised against recombinant Pf TyrRS. Our localization data show that Pf TyrRS is present in all three stages of asexual parasite life cycle: rings, trophozoites and schizonts ( Fig. 3a ; Supplementary Movies 1 , 2 and 3 based on z-stacked confocal analyses of rings, trophozoites and schizonts, respectively—DAPI is in blue and Pf TyrRS in green). Closer examination of Pf TyrRS localization in infected erythrocytes during trophozoite and schizont stages revealed possible secretion of Pf TyrRS into infected red blood cell (iRBC), despite absence of an export signal in Pf TyrRS sequence ( Fig. 3a ). Similar results were obtained using Pf TyrRS-GFP fusion parasite transgenic cell lines ( Fig. 3b ). We therefore tested whether secretion of Pf TyrRS occurred from schizonts at time of iRBC rupture. To address this, culture supernatants of infected RBCs were separated on SDS–PAGE, and western blotting was performed using anti- Pf TyrRS antisera ( Fig. 3c ). This experiment indicated a band of ∼ 42 kDa in iRBC medium that corresponds to the molecular size of Pf TyrRS. As controls, the parasite-secreted MSP1 and non-secreted proteins like DTD [32] , [33] and falcipain 2 were also used ( Fig. 3c ). We also performed western blot analysis using anti-GFP antibody on Pf TyrRS-GFP parasite cell line supernatants. Pf TyrRS-GFP fusion protein band of expected molecular weight (70 kDa) was clearly seen in iRBCs supernatants but not in supernatants from uninfected RBCs controls ( Fig. 3d ). These experiments suggest that Pf TyrRS is expressed in all asexual parasite stages, and that it is exported to the host erythrocyte cytosol, from where it is released into blood plasma on iRBC rupture. 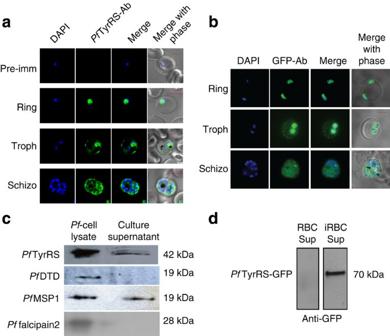Figure 3: Cellular localization ofPfTyrRS. (a) Confocal microscopy ofP. falciparumasexual stages—rings, trophozoites and schizonts using anti-sera raised in rabbits againstPfTyrRS. Scale bar in red corresponds to a size of 5 μm (b) Confocal microscopy using anti-GFP antibody (green) inPfTyrRS-GFP transgenic parasite cell lines. Parasite nucleus was stained with DAPI (blue) in each case. Scale bar in red corresponds to a size of 5 μm. (c) Enhanced chemi-luminiscence of parasite culture supernatants using antibodies againstPfTyrRS,PfDTD,PfMSP1 andPffalcipain 2 and (d) Enhanced chemi-luminiscence of parasite culture supernatants using anti-GFP antibody. Figure 3: Cellular localization of Pf TyrRS. ( a ) Confocal microscopy of P. falciparum asexual stages—rings, trophozoites and schizonts using anti-sera raised in rabbits against Pf TyrRS. Scale bar in red corresponds to a size of 5 μm ( b ) Confocal microscopy using anti-GFP antibody (green) in Pf TyrRS-GFP transgenic parasite cell lines. Parasite nucleus was stained with DAPI (blue) in each case. Scale bar in red corresponds to a size of 5 μm. ( c ) Enhanced chemi-luminiscence of parasite culture supernatants using antibodies against Pf TyrRS, Pf DTD, Pf MSP1 and Pf falcipain 2 and ( d ) Enhanced chemi-luminiscence of parasite culture supernatants using anti-GFP antibody. Full size image Pf TyrRS interaction with host immune cells Release of Pf TyrRS from iRBCs and the presence of an exposed and conformationally competent ELR motif persuaded us to address directly the binding of TyrRS to host immune cells. We performed an in vivo experiment where mice were infected with Plasmodium yoelii (XNL). Subsequently, spleen cells containing peripheral blood mononuclear cells (PBMCs) were isolated from these infected mice and then presence of native TyrRS was tested using anti-TyrRS-specific antibodies by flow cytometry ( Fig. 4a ). We observed specific TyrRS binding to mouse macrophages and dendritic cells, among others ( Fig. 4a ). A corresponding in vitro experiment using human PBMCs also showed specific interaction of Pf TyrRS with human macrophages and, to a lesser degree, with dendritic cells ( Fig. 4b ). To validate these observations further, we assessed binding of Pf TyrRS to mouse and human immune cells using confocal microscopy ( Fig. 4c,d ). We detected both binding and internalization of Pf TyrRS by host macrophages. Supplementary Movie 4 is based on Z-stacking of these confocal images where macrophages are stained for nucleus (DAPI, blue) and for Pf TyrRS (in green). These data led us to hypothesize an ELR-motif-mediated interaction of P. falciparum tyrosyl-tRNA synthetase with human macrophages ( Fig. 4c,d ). 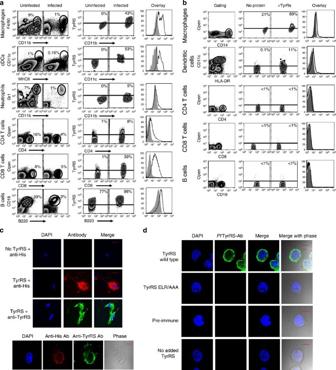Figure 4: TyrRS interaction with PBMCs in vivoandin vitro. (a) FACS-based binding of mouse PBMCs with anti-PfTyrRS antibodies in anex vivoexperiment. Left panel shows gating; middle panel shows TyrRS binding in immune cells tested in both uninfected and infected mice. Overlay histograms are derived from the TyrRS expression dot plots wherein solid grey histogram is uninfected and the black bold line represents data for infected mice. Data are cumulative of two independent experiments. (b) Binding ofPfTyrRS to human PBMCs showing specific interaction with human macrophages and dendritic cells. Left panel shows gating; middle panel showsPfTyrRS binding to various immune cells. The overlay histogram is derived fromPfTyrRS-binding dot plots wherein solid grey histogram is withoutPfTyrRS and black solid line is withPfTyrRS. Confocal images of binding and internalization ofPfTyrRS into (c) mouse dendritic cells (top panel), mouse macrophages (bottom panel) and (d) human macrophages. In (d) along with wild-typePfTyrRS (green), the controls of pre-immune sera, ELR/AAA mutantPfTyrRS, and primary/secondary antibodies alone (that is, no addedPfTyrRS) are shown. For nucleus visualization, DAPI (blue) localization is also shown. The red scale bar in confocal images corresponds to a size of 15 μm. Figure 4: TyrRS interaction with PBMC s in vivo and in vitro . ( a ) FACS-based binding of mouse PBMCs with anti- Pf TyrRS antibodies in an ex vivo experiment. Left panel shows gating; middle panel shows TyrRS binding in immune cells tested in both uninfected and infected mice. Overlay histograms are derived from the TyrRS expression dot plots wherein solid grey histogram is uninfected and the black bold line represents data for infected mice. Data are cumulative of two independent experiments. ( b ) Binding of Pf TyrRS to human PBMCs showing specific interaction with human macrophages and dendritic cells. Left panel shows gating; middle panel shows Pf TyrRS binding to various immune cells. The overlay histogram is derived from Pf TyrRS-binding dot plots wherein solid grey histogram is without Pf TyrRS and black solid line is with Pf TyrRS. Confocal images of binding and internalization of Pf TyrRS into ( c ) mouse dendritic cells (top panel), mouse macrophages (bottom panel) and ( d ) human macrophages. In ( d ) along with wild-type Pf TyrRS (green), the controls of pre-immune sera, ELR/AAA mutant Pf TyrRS, and primary/secondary antibodies alone (that is, no added Pf TyrRS) are shown. For nucleus visualization, DAPI (blue) localization is also shown. The red scale bar in confocal images corresponds to a size of 15 μm. Full size image Triggering of cytokine secretion by Pf TyrRS Our observations on interaction of Pf TyrRS with host immune cells prompted us to test whether the ELR motif present in Pf TyrRS could enable it to trigger release of cytokines from macrophages. We tested this hypothesis by incubating mouse and human macrophage cell lines with recombinant wild-type Pf TyrRS, with a mutant ELR/AAA- Pf TyrRS, with lipopolysaccharide (LPS) (as positive control), with media alone and PfDTD (last two as negative controls). In these studies, the amounts of Pf TyrRS used were in nanomolar (nM) concentration ranges, similar to amounts used in studies with human mini-TyrRS [9] , [10] , [11] , [12] , [13] . Time kinetic analysis using ELISA revealed maximal production of the inflammatory cytokines TNF-α, IL-6 and IL-1(α and β) within 6 hours of culture (Tukey's test— P <0.001) ( Fig. 5a,b ), but not of IL-10 or IL-12 ( Fig. 5c ). The cytokine release mediated by Pf TyrRS was dose-dependent, and occurred as early as 4 hours post-incubation of macrophages with Pf TyrRS ( Fig. 5d ). Interestingly, the mutant Pf TyrRS (where ELR was replaced with AAA sequence) did not trigger cytokine release from macrophages and behaved similar to the control proteins Pf DTD [32] , [33] or Pf SerRS. In all experiments, LPS was used as a positive control, and all proteins used in these experiments were confirmed to be endotoxin free (Methods). We also observed that Pf TyrRS that had been immunoprecipitated from parasite culture supernatants was equally capable of triggering release of TNF-α and IL-6 from human macrophage ThP1 cell lines ( Fig. 5e ). Finally, pre-incubation of Pf TyrRS with anti- Pf TyrRS antibodies substantially blocked TNF-α (Tukey's test— P <0.05) and IL-6 production (Tukey's test— P <0.01) from human macrophages ( Fig. 5e ), suggesting specific, motif-based Pf TyrRS interaction with human macrophages. 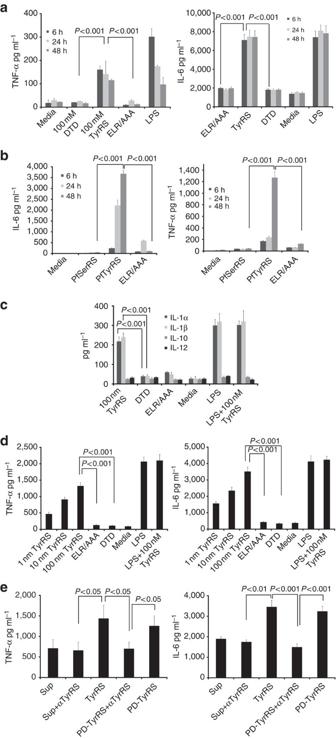Figure 5: Effect ofPfTyrRS on mouse macrophages. (a) Cytokines levels were measured using BioPlex kit (Bio-Rad) and the secretion profiles of TNF-α and IL-6 using mouse macrophages were measured at different time points. Media alone,PfDTD/PfSerRS enzymes and ELR-AAA mutant ofPfTyrRS were used as negative controls. LPS was used as positive control in all experiments. (b) Identical experiment as in (a) except that the human macrophage cell line ThP1 was used. This experiment has the extra negative control ofPfSerRS. (c) Secretion profiles of extra cytokines (IL-1, IL-10 and IL-12) that are secreted from human macrophages on exposure toPfTyrRS. (d) Dose-dependent increase in secretion of TNF-α and IL-6 when increasing concentrations ofPfTyrRS were used with human macrophages. (e) Cytokine secretion profiles usingP. falciparumculture supernatants alone (Sup), supernatants incubated with anti-TyrRS antibody (Sup+αTyrRS), parasite culture supernantant-immunoprecipitatedPfTyrRS (PD-TyrRS) and finally parasite culture supernantant -immunoprecipitatedPfTyrRS with its antibody (PD-TyrRS + αTyrRS). TNF-α and IL-6 secretion is clearly enhanced significantly when immunoprecipitatedPfTyrRS (PD-TyrRS) is used. Triggering activity ofPfTyrRS (PD-TyrRS) is blocked when pre-incubated with anti-PfTyrRS antibodies, indicating specific activation of macrophages with nativePfTyrRS (PD-TyrRS). Experiments were repeated three times and error bars indicate standard deviation. Tukey's test was performed andP-values are shown such that the end points of the lines belowP-value represent the datasets that were compared. Figure 5: Effect of Pf TyrRS on mouse macrophages. ( a ) Cytokines levels were measured using BioPlex kit (Bio-Rad) and the secretion profiles of TNF-α and IL-6 using mouse macrophages were measured at different time points. Media alone, Pf DTD/ Pf SerRS enzymes and ELR-AAA mutant of Pf TyrRS were used as negative controls. LPS was used as positive control in all experiments. ( b ) Identical experiment as in ( a ) except that the human macrophage cell line ThP1 was used. This experiment has the extra negative control of Pf SerRS. ( c ) Secretion profiles of extra cytokines (IL-1, IL-10 and IL-12) that are secreted from human macrophages on exposure to Pf TyrRS. ( d ) Dose-dependent increase in secretion of TNF-α and IL-6 when increasing concentrations of Pf TyrRS were used with human macrophages. ( e ) Cytokine secretion profiles using P. falciparum culture supernatants alone (Sup), supernatants incubated with anti-TyrRS antibody (Sup+αTyrRS), parasite culture supernantant-immunoprecipitated Pf TyrRS (PD-TyrRS) and finally parasite culture supernantant -immunoprecipitated Pf TyrRS with its antibody (PD-TyrRS + αTyrRS). TNF-α and IL-6 secretion is clearly enhanced significantly when immunoprecipitated Pf TyrRS (PD-TyrRS) is used. Triggering activity of Pf TyrRS (PD-TyrRS) is blocked when pre-incubated with anti- Pf TyrRS antibodies, indicating specific activation of macrophages with native Pf TyrRS (PD-TyrRS). Experiments were repeated three times and error bars indicate standard deviation. Tukey's test was performed and P -values are shown such that the end points of the lines below P -value represent the datasets that were compared. Full size image Potential receptor(s) for Pf TyrRS on human macrophages To identify a receptor for Pf TyrRS on macrophages, we pre-incubated human macrophages with anti-CXCR1/2 and anti- Pf TyrRS antibodies, and tested whether antibody-mediated receptor or protein blockades inhibited Pf TyrRS-macrophage interaction ( Fig. 6a ). Specific antibody-mediated blocking of CXCR2 receptor (Tukey's test— P <0.05), but not the CXCR1 receptor, on human macrophages reduced Pf TyrRS binding by ∼ twofold ( Fig. 6a ). Blocking of Pf TyrRS with anti- Pf TyrRS antibodies also reduced binding of the protein to macrophages (Tukey's test— P <0.05) ( Fig. 6a ). Furthermore, blockage of Pf TyrRS-macrophage interactions using either anti-CXCR2 or anti- Pf TyrRS antibodies also significantly reduced the release of TNF-α (Tukey's test— P <0.05) and IL-6 (Tukey's test— P <0.001) from human macrophages ( Fig. 6b ). To further probe the significance of ELR motif in binding of Pf TyrRS to macrophages, we tested inhibition of Pf TyrRS-macrophage interaction using peptides in which the wild-type Pf TyrRS ELR peptide sequence (D ELR V) was mutated residue-wise to DEL A V, D AAA V and DEL K L. Fluorescence-activated cell sorting (FACS)-based binding studies of Pf TyrRS in presence of 100 nM of these peptides showed a significant reduction in binding with only the D ELR V peptide sequence ( Fig. 6c ). The DEL K L peptide was less competent in competing whereas the other two peptides did not compete at all ( Fig. 6c ). Additionally, the Pf TyrRS-triggered release of TNF-α and IL-6 from human macrophages was significantly reduced in presence of D ELR V peptide (Tukey's test— P <0.05) ( Fig. 6d ). These data, along with our observation that the 'ELR/AAA' Pf TyrRS mutant does not bind to human macrophage cells ( Fig. 4c,d ), strongly highlight a role for ELR motif in Pf TyrRS interactions with human macrophages. We therefore conclude that ELR-motif-based Pf TyrRS binding likely occurs using specific receptors on human macrophages, and that this binding leads to very specific host immune system activation. 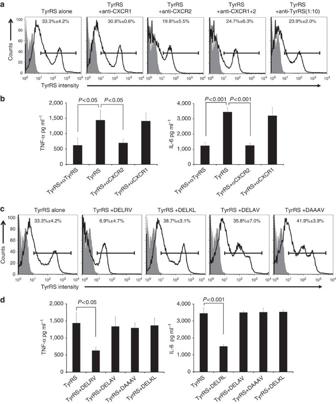Figure 6: PotentialPfTyrRS receptor on human macrophages. (a) FACS analysis ofPfTyrRS binding to human macrophages.PfTyrRS binding to macrophages is reduced when macrophages had been pre-incubated anti-CXCR2 or with anti-PfTyrRS antibodies. Binding was not reduced significantly with anti-CXCR1 antibodies. Overlay histograms show binding ofPfTyrRS to the surface of human macrophages (black line) with unstained controls (grey solid) as background. (b) Cytokine secretion assays for TNF-α and IL-6 using human macrophages and anti-CXCR1, anti-CXCR2 and anti-PfTyrRS antibodies. Secretion of these pro-inflammatory cytokines is reduced when anti-CXCR2 and anti-PfTyrRS antibodies were pre-incubated with human macrophages. (c) FACS analysis ofPfTyrRS binding to human macrophages using four different ELR-mutant peptides in competition assays. Overlay histograms showPfTyrRS surface staining (black line) with unstained control (grey solid) as background. (d) Cytokine secretion assays for TNF-α and IL-6 using human macrophages and various ELR-mutant peptides. No significant difference was observed for mutant peptides in these assays. Experiments were repeated three times and the error bars indicate the standard deviation. Tukey's test was performed andP-values are shown such that the end points of the lines belowP-value represent the datasets that were compared. Figure 6: Potential Pf TyrRS receptor on human macrophages. ( a ) FACS analysis of Pf TyrRS binding to human macrophages. Pf TyrRS binding to macrophages is reduced when macrophages had been pre-incubated anti-CXCR2 or with anti- Pf TyrRS antibodies. Binding was not reduced significantly with anti-CXCR1 antibodies. Overlay histograms show binding of Pf TyrRS to the surface of human macrophages (black line) with unstained controls (grey solid) as background. ( b ) Cytokine secretion assays for TNF-α and IL-6 using human macrophages and anti-CXCR1, anti-CXCR2 and anti- Pf TyrRS antibodies. Secretion of these pro-inflammatory cytokines is reduced when anti-CXCR2 and anti- Pf TyrRS antibodies were pre-incubated with human macrophages. ( c ) FACS analysis of Pf TyrRS binding to human macrophages using four different ELR-mutant peptides in competition assays. Overlay histograms show Pf TyrRS surface staining (black line) with unstained control (grey solid) as background. ( d ) Cytokine secretion assays for TNF-α and IL-6 using human macrophages and various ELR-mutant peptides. No significant difference was observed for mutant peptides in these assays. Experiments were repeated three times and the error bars indicate the standard deviation. Tukey's test was performed and P -values are shown such that the end points of the lines below P -value represent the datasets that were compared. Full size image Pf TyrRS-stimulated macrophage upregulate ICAM-1 and VCAM-1 P. falciparum cytoadherence enables parasite sequestration in host tissues, allowing these parasites to avoid splenic clearance which involves degradation and clearing of infected RBCs by the spleen [34] , [35] , [36] , [37] , [38] , [39] , [40] . In severe malaria episodes, an increase in the levels of TNF-α is coupled with enhanced expression of endothelial cell receptors such as ICAM-1 (intercellular adhesion molecule-1), VCAM-1 (vascular cell adhesion molecule-1) and E-selectin [34] , [35] , [36] , [37] , [38] , [39] , [40] . We therefore tested whether recombinant Pf TyrRS could modulate expression of endothelial receptors in a static cytoadhesion model assay system. For this 'triggering' to work, Pf TyrRS had to first initiate enhanced secretion of cytokines like TNF-α from macrophages, and then the increased levels of secreted cytokines would have to induce overexpression of endothelial receptors like ICAM-1 and VCAM-1. As our experimental data show, this is indeed what Pf TyrRS was able to achieve ( Fig. 7 ). When HUVECs (primary human umbilical vein endothelial cells) were co-cultured with culture supernatants of Pf TyrRS-activated macrophages, we found strong upregulation of both ICAM-1 and VCAM-1 receptors (Tukey's test— P <0.05) ( Fig. 7a ). A Pf TyrRS-induced dose-dependent increase in expression of ICAM-1 was also evident ( Fig. 7b ). These effects were not due to cell toxicity of Pf TyrRS on HUVECs ( Fig. 7c ). These experiments therefore provide fundamental molecular insights and also a tool to dissect the molecular basis of cytoadherence using Pf TyrRS as a 'trigger'. Increased levels of circulating cytokines in malaria infected individuals may activate the host immune system to check or control very high parasitemia levels, which may prove lethal both to pathogen and host. 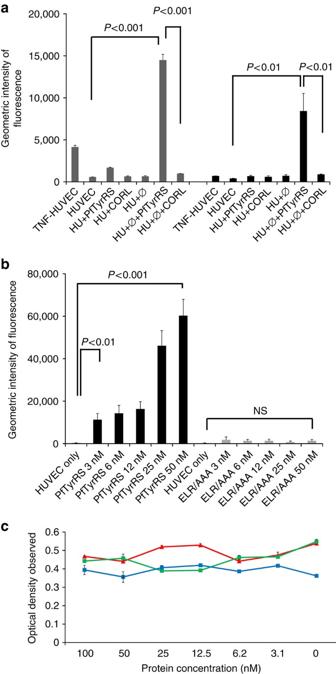Figure 7:PfTyrRS stimulation of macrophages and subsequent upregulation of endothelial receptors ICAM-1 and VCAM-1. (a) HUVEC cells (Hu) were incubated withPfTyrRS alone,PfDTD (negative control protein (CORL), macrophage cells (φ) and TNF-α. Culture supernatants ofPfTyrRS-induced macrophages andPfDTD-induced macrophages were added to HUVEC cell lines. Expression of ICAM-1 and VCAM-1 was measured by FACS using specific conjugated antibodies. Grey bars (left) represent VCAM-1 expression and black bars (right) represent ICAM-1 expression. (b)PfTyrRS-induced dose-dependent increase in the expression of ICAM-1. No upregulation of ICAM-1 was observed on addition of ELR/AAAPfTyrRS mutant to endothelial cell lines. Bars in black representPfTyrRS treated samples, whereas bars in grey were the samples treated with ELR/AAA mutant protein (c) MTT cytotoxicity assay with dose-dependent response usingPfTyrRS (red line), ELR/AAA mutant (green line), and control (only cells in blue line) on HUVEC cells. No decrease in cell viability was observed (Tukey's test—P>0.05). The optical density onyaxis in (c) represents cell survival in an MTT assay. Experiments were repeated three times and the error bars represent standard deviation. Tukey's test was performed andP-values are shown such that the end points of the lines belowP-value represent the datasets that were compared. NS, not significant. Figure 7: Pf TyrRS stimulation of macrophages and subsequent upregulation of endothelial receptors ICAM-1 and VCAM-1. ( a ) HUVEC cells (Hu) were incubated with Pf TyrRS alone, Pf DTD (negative control protein (CORL), macrophage cells (φ) and TNF-α. Culture supernatants of Pf TyrRS-induced macrophages and Pf DTD-induced macrophages were added to HUVEC cell lines. Expression of ICAM-1 and VCAM-1 was measured by FACS using specific conjugated antibodies. Grey bars (left) represent VCAM-1 expression and black bars (right) represent ICAM-1 expression. ( b ) Pf TyrRS-induced dose-dependent increase in the expression of ICAM-1. No upregulation of ICAM-1 was observed on addition of ELR/AAA Pf TyrRS mutant to endothelial cell lines. Bars in black represent Pf TyrRS treated samples, whereas bars in grey were the samples treated with ELR/AAA mutant protein ( c ) MTT cytotoxicity assay with dose-dependent response using Pf TyrRS (red line), ELR/AAA mutant (green line), and control (only cells in blue line) on HUVEC cells. No decrease in cell viability was observed (Tukey's test— P >0.05). The optical density on y axis in ( c ) represents cell survival in an MTT assay. Experiments were repeated three times and the error bars represent standard deviation. Tukey's test was performed and P -values are shown such that the end points of the lines below P -value represent the datasets that were compared. NS, not significant. Full size image One of the key pathogenic mechanisms in the virulence of P. falciparum is the phenomenon of cytoadherence, attributed to increased adhesion of infected erythrocytes to blood capillaries [34] , [35] , [36] , [37] , [38] , [39] , [40] , [41] , [42] . In particular, cerebral and placental malaria seem to be dependent on crucial protein–protein interactions that occur between a parasite virulence factors and the endothelial/placental receptors [34] , [35] , [36] , [37] , [38] , [39] , [40] , [41] , [42] . The host immune system is hijacked by parasite-derived factors to assist in cytoadherence, for example, by cytokine-induced increased expression of a range of adhesion molecules [16] , [18] , [19] , [20] , [21] , [22] , [23] , [24] , [25] . Numerous field reports on human malaria and mouse model studies have shown that malaria infection alters host cytokine profiles by modulating dendritic cells and macrophages [16] , [18] , [19] , [20] , [21] , [22] , [23] , [24] , [25] . This is presumably done to aid in parasite survival and transmission. Elevated cytokine levels have a variety of physiological effects, generally to the detriment of the hosts [16] , [34] , [35] , [36] , [37] , [38] , [39] , [40] , [41] , [42] . In fact, malaria as a disease has been looked up on as a manifestation of enhanced pro-inflammatory cytokine production in host [16] , [34] , [35] , [36] , [37] , [38] , [39] , [40] , [41] , [42] . For example, the clinical manifestations of severe malaria can be correlated with induction of strong pro-inflammatory responses in which plasma levels of circulating TNF-α, IFN-γ and IL-6 increase significantly [19] , [20] , [21] . Pathways that propel host immune cell activation in malaria remain mysterious in context of parasite-derived protein antigens. The interaction of latter with macrophages and dendritic cells must occur before cytokine induction. So far, studies have identified several such molecular agents [2] , [3] , [4] , [5] , [6] , [7] , [8] , [9] , [10] , [11] , [12] , [13] , [14] , [15] , [16] , [17] , [18] , [19] , [20] , [21] , [22] , but, to our knowledge, no parasite-secreted housekeeping enzyme has been attributed with the ability to trigger enhanced secretion of cytokines like TNF-α and IL-6. In this context, we find it very interesting that the levels of TNF-α secreted from immune cells reported in previous studies [22] , [23] , [24] , [25] are similar to or lower than those we report with Pf TyrRS. A comparison of secreted TNF-α levels (pg ml −1 ) is illuminating—using 100 nM Pf TyrRS: 1,000–1,300 pg ml −1 , 50–400 nM GPIs; 800–1,300 pg ml −1 , ∼ μg ml −1 DNA-protein complexes; 500–600 pg ml −1 and 30–100 μM hemozoin; 400–600 pg ml −1 , ∼ 500,000 microparticles; 150–200 pg ml −1 . This comparison indicates importance of Pf TyrRS as a trigger for excitation of pro-inflammatory cytokine release from host immune cells. Our corroborative confocal microscopy data not only reveals decoration of host macrophage surfaces with Pf TyrRS but also its internalization. We propose that, as a result of Pf TyrRS-macrophage interactions, significantly higher amounts of pro-inflammatory cytokines like TNF-α, IL-1 and IL-6 are released. Elevated cytokine levels can have severe effects in hosts and severe malarial anemia (SMA) provides an excellent example of this [45] . Increased circulating TNF-α inhibits erythroblast differentiation and dampens erythropoiesis resulting in worsening SMA symptoms [16] , [17] , [18] , [19] , [20] , [21] , [45] . Another outcome of higher levels of circulating TNF-α in infected malaria patients is the increase in expression levels of certain endothelial receptors like ICAM-1, VCAM-1 and E-selectin that contribute to cytoadherence in severe malaria [39] , [40] , [41] , [42] . Our data based on co-incubation of three components—purified Pf TyrRS macrophages and endothelial cells, now provides a system that can be further dissected to investigate molecular and cellular interactions that occur during SMA and cytoadherence. This work therefore provides clues to the possibility of Pf TyrRS acting as a malarial toxin that can induce cytokine-mediated disease. Aminoacyl-tRNA synthetases have a vital role in translating the genetic code. Numerous studies have shown that members of this enzyme family are quite adept at 'moonlighting' in terms of possessing extra capabilities that widen their biological attributes [5] , [6] , [7] , [8] . Studies have indicated that human tyrosyl-, tryptophanyl- and lysyl-tRNA synthetases can be secreted extracellularly and can mimic cytokines [5] , [6] , [7] , [8] . For these extra roles, the human TyrRS and TrpRS require either proteolytic cleavage or alternate splicing to become active [5] , [6] , [7] , [8] , [9] , whereas LysRS can act like a cytokine without processing [44] . In this light, this is the first report of a human pathogen tRNA synthetase that can also perform moonlighting activity of inducing host immune system to release pro-inflammatory cytokines. In summary, this study suggests that Pf TyrRS is secreted from the parasite and deposited proximal to iRBC membrane (despite lack of a 'PEXEL' export element [43] ). Pf TyrRS egress occurs during trophozoite and schizont stages, before iRBC rupture. On iRBC lysis, Pf TyrRS is released into blood plasma, where it is potentially free to interact with host cells. We show that Pf TyrRS interacts with specific receptor(s) on host macrophages, and that this event is largely mediated by the ELR motif present in Pf TyrRS. Finally, we have determined the three-dimensional structure of Pf TyrRS in complex with Tyr-AMP, and provide detailed structural comparisons with host counterpart of Pf TyrRS. This work therefore not only provides a structural framework for using Pf TyrRS-YAP complex structure as a starting point for structure-based drug discovery, but also lays foundation for probing key immunological questions in malaria. The twin abilities of malaria parasite tyrosyl-tRNA synthetase—as a housekeeping protein translation enzyme and as a trigger for pro-inflammatory cytokine release in hosts—highlight this protein as a target for discovery of novel anti-parasitic strategies. Animal experiments Animal experiments were performed in accordance with Institutional Animal Ethics Committee guidelines approved by Department of Biotechnology, Govt of India. This project was approved in a meeting held on 28 October 2009 at ICGEB (approval ID: ICGEB/IAEC/MAL-50). All mice used were killed ethically by asphyxiation in carbon dioxide according to regulatory body instructions. Synthetic tRNA preparation and aminoacylation assay Synthetic Plasmodium falciparum tRNA clones were obtained according to Sampson and Uhlenbeck [46] by assembling up to 6 oligonucleotides and ligation between HindIII and BamHI sites into pUC19 vector. The tRNAs were obtained by in vitro transcription using T7 RNA polymerase according to standard protocols. In vitro tRNA aminoacylation assays were performed at 37 °C in 50 mM Tris–HCl pH 7.6, 50 mM KCl, 25 mM MgCl 2 , 5 mM ATP, 0.1 mg ml −1 BSA, 1 mM DTT, 20 μM tyrosine, 0.5 mCi ml −1 L –[3,5-3H]tyrosine and 0.5 μM Pf TyrRS as reported [47] . Reaction was initiated by addition of pure enzyme and samples of 20 μl were spotted onto Whatman 3 mM discs at varying time intervals (usually 2 min). Radioactivity (corresponding to amino acid ligated to tRNA substrate) was measured by liquid scintillation. Protein expression, purification and crystallization TyrRS gene (MAL8P1.125). from P. falciparum was PCR amplified from complementary DNA and cloned into pQE30 vector (Qiagen). Four hours post -IPTG (isopropyl 1-thio- D -galactopyranoside, 0.5 mM) induction, the bacterial cell pellet was suspended in buffer containing 50 mM Tris–HCl, 500 mM NaCl, 50 mM imidazole, pH 8.0 and protease inhibitor cocktail. Protein was purified using Ni-NTA beads (Qiagen) and gel filtration chromatography. Pure, dimeric Pf TyrRS was concentrated and buffer exchanged into 25 mM Tris–HCl pH 8.0, 150 mM NaCl and 10 mM BME. Diffraction quality crystals using His-tag-free Pf TyrRS were grown by hanging drop vapour diffusion method at 20 °C. The droplet size was 1 μl of protein (30 mg ml −1 in 25 mM Tris pH 8.0, 100 mM NaCl, 10 mM BME, 10 mM MgCl 2 , 10 mM ATP and 2 mM L –tyrosine) with 1 μl of reservoir solution equilibrated over 200 μl of 2.4 M sodium malonate at pH 6.0. Data collection and structure determination A single crystal was transferred to cryoprotectant reagent (paratone oil) for a short period (5–10 s) before freezing in a stream of cooled nitrogen gas. Data were collected at 100 K using Cu Kα radiation ( λ =1.54 Å) on a MAR345 image-plate detector mounted on a Rigaku MicroMax-007 rotating-anode X-ray generator. A total of 700 frames were collected in 1° oscillation steps with 5 min exposure per frame, and data were processed with HKL2000 (ref. 48 ). The structure was solved by molecular replacement in MOLREP [49] using cytoplasmic mini-HsTyrRS (PDB: 1N3L ) as a starting model. Iterated manual model building and refinement was done using COOT [50] and phenix.refine [51] . The structural representations in this paper were prepared with Chimera [52] and PyMOL ( http://www.pymol.org ). Cell-binding assays For in vitro localization experiments, synchronous parasite cultures of P. falciparum 3D7 were washed with PBS, fixed in solution using 4% paraformaldehyde and 0.0075% glutraldehyde for 20 min, permeablized with 0.1% Triton X-100 for 10 min and then treated for 10 min with 0.1 mg ml −1 sodium borohydride in PBS. Each step was followed by a brief PBS wash [53] . Cells were blocked in 3% BSA, PBS for 1 h, washed in PBS and incubated overnight with protein-A column purified rabbit anti- Pf TyrRS antibodies (1:150 dilution in PBS containing 3% BSA) at 4 °C. After three washes (10 min each) with PBS, the cells were incubated with Alexa Fluor 488 -conjugated anti-rabbit secondary antibody (1:250 dilution in PBS containing 3% BSA) for 2 h at room temperature and allowed to settle onto poly- D -lysine (100 mg ml −1 )-coated coverslips. These were then washed three times in PBS and mounted in antifade with DAPI (Molecular Probes). Spleen cells were purified from P. yoelii -infected mice and PBMCs were isolated from both mouse and human blood as described earlier [54] . For the in vivo experiment, C57BL/6 mice were infected with ∼ 1 million P . yoelii (17XNL strain) in the form of parasitized RBC's intraperitoneally. Fifteen days after infection, the spleens were collected from infected and age-and-sex matched uninfected control mice. Spleens were crushed and lymphocytes were isolated and stained for flow cytometry by standard procedures. The cells were fixed with Cytofix (BD Biosciences) and permeabilized with 1X Cytoperm (BD Biosciences) for intracellular TyrRS staining. The data was acquired on BD FACS Canto II (BD Biosciences) and analysed on by FlowJo software (Treestar). Human PBMCs were isolated using BD Vacutainer CPT tubes (BD Biosciences) by centrifugation at 1,600 g per 25 min/RT/no brake. The cells were thoroughly washed and resuspended in complete RPMI containing 10% FCS in a 24-well plate, and 100 nM purified Pf TyrRS protein was added for 3 h at 37 °C (95% humidity, 5% CO 2 ). Analytical flow cytometry was performed by direct staining for specific populations of immune cells with fluorescently conjugated antibodies and biotin-conjugated anti- Pf TyrRS antibody (1:150 dilution in PBS). The data obtained on BD FACS Canto II (BD Biosciences) was analysed using FlowJo software (Treestar). In vitro binding of Pf TyrRS to various immune cells was performed by FACS using standard protocols. Dendritic cells and macrophage ThP1 cells were cultured on coverslips in 24-well plates (Gibson) and maintained in DMEM medium containing 20% (v/v) FBS and 1% antibiotics (Gibco). Pf TyrRS and other control proteins were incubated with cells at several concentrations for 5 min to 2 h at 4 °C. Cells were washed twice in PBS and incubated with 2% formaldehyde (Sigma) for 15 min and followed by incubation for 10 min with 0.1% saponin (Sigma). Primary and secondary antibodies were added as per manufacturer's instructions (Molecular Probes). Fluorescence microscopy was performed on Nikon A1R confocal laser scanning microscope. Western blots P. falciparum (schizont stage) -infected human erythrocytes (1.5×107 parasites per ml) were enriched and parasites were cultured for 6–10 h to allow the maturation of schizonts, release of merozoites and their material [54] . Culture supernatant was collected in the presence of protease inhibitor cocktail after two rounds of centrifugation of 1,000 g for 15 min followed by 10,000 g for 20 min before freezing at −70 °C. Culture supernatant was subsequently used for western blotting using different antibodies against Pf DTD (dilution, 1:500), Pf falcipain 2 (dilution, (1:1,000), Pf MSP-1 (dilution, 1:1,000) and Pf TyrRS (dilution, 1:500). Cytokine secretion assays Raw-264.7. cells, J774 murine cells, Dendritic cells (isolated from femur bone marrow of the mice C57BL/6) and human THP1 macrophage cells (3×10 4 ) were cultured in RPMI medium with 10% FBS and 1% antibiotics in 24-well format plates. Proteins were passed through polymyxin beads (Sigma) before assays. LPS, Pf TyrRS and control proteins were added to the medium at different concentrations. 100 μl of culture medium was collected and centrifuged after every 4, 24 and 48 h. Cytokines in the culture supernatant were detected by a Luminex microbead-based multiplexed assay (Bio-Plex manager 5.0) using commercially available kits according to the manufacturer's protocol (Bio-Plex, Bio-Rad). All proteins were tested for endotoxin contaminations and passed through polymyxin beads (Sigma). LAL (Limulus Amebocyte Lysate) assay was performed to confirm that the proteins were endotoxin-free before each assay. Pf TyrRS interaction with human macrophages Cultured human macrophages cells were mixed with Pf TyrRS in absence or presence of different antibodies, namely anti- Pf TyrRS, anti-CXCR1 and anti-CXCR2. Binding of Pf TyrRS was tested using standard FACS protocols. In related experiments, cytokine profiling of these human macrophages was also done, either in absence or presence of antibodies used above. Cytokines released in culture supernatants were detected by a Luminex microbead-based multiplexed assay (Bio-Plex manager 5.0) using commercially available kits and according to the manufacturer's protocol (Bio-Plex, Bio-Rad). Similar experiments were performed using various wild-type and mutant ELR-based peptides. Human macrophages (ThP1 cells) were incubated with 100 nM of these peptides before addition of Pf TyrRS. FACS and cytokine profiling were again done on all these samples as for the antibody treatment experiments. Upregulation of endothelial cell receptors Monocytes were obtained from buffy coat by Lymphoprep (Axis-Shield) gradient centrifugation, followed by adhesion-mediated purification on tissue culture plastic. The cells were cultured for 3 days in RPMI-164 medium (Sigma) supplemented with 2 mM L -glutamine and 10% FBS to differentiate into macrophage. The recombinant Pf TyrRS or control proteins were added at a concentration of 1 μl ml −1 on day 3, and cells were cultured continuously for 3 days. The culture supernatant was collected and centrifuged at 13,000 g for 10 min to remove any debris; the supernatant was used for co-culture with endothelium. Primary pooled human umbilical vein endothelial cells (HUVEC) were obtained from Promocell). Cells were maintained in complete growth medium supplied by Promocell, according to the company's instructions. To reduce variation, only cells at passage five to six were used. HUVEC were grown on 1% gelatin (Sigma) coated on 24-well plates with appropriate growth medium, until confluent. Then, the culture medium was replaced with either fresh medium alone, medium containing recombinant Pf TyrRS or control protein (added at concentration 100 nM) or macrophage culture supernatants. These were incubated at 37 °C in 5% CO 2 for 16 h. Endothelial cell markers were measured by fluorescence-activated cell sorting (FACScan; Becton Dickinson). Specific fluorescence-conjugated antibodies, including APC Mouse anti-human CD54 (ICAM-1) and PE Mouse anti-human CD106 (VCAM-1) (Becton Dickinson), were used in this study. Nonspecific fluorescence was assessed using corresponding isotype control antibodies. The expression of endothelial surface proteins ICAM-1 and VCAM-1 was indicated by geometric mean of the fluorescence intensity. Pf TyrRS was subsequently used in a dose-dependent experiment for testing increased expression of ICAM-1, using the protocols described above. Pf TyrRS-GFP microscopy The gene was amplified with genomic DNA of P. falciparum using following primers: forward-5′-CTCGAGATGATAATATTAAAGGTTTTATTTA-3′ reverse-5′-GGTACCTTTTATTATTATAGAATAACTTGTTC-3′ and cloned into pGEM-T vector (Promega). The insert was released from pGEMT and cloned between XhoI and KpnI in pGlux vector (Amersham). Transformations and clone propagation was done in Dh5α cells. Transfection of vectors into the parasite was done, as described earlier [55] . GFP-expressing infected erythrocytes were studied live or fixed at ambient temperature. Cells were viewed with a UPlanSApo ×100 1.4 oil objective on a Olympus IX81 Live Cell Imaging Inverted Microscope equipped with an Olympus F-View camera and primarily processed with analySIS LS Research software package. Captured images were then further processed using Photoshop and ImageJ. Pictures were adjusted to gain optimal contrast to visualize features of interest. MTT assays HUVEC cells at passage 5 were seeded at a concentration of 2×10 4 cells per well (in 100 μl) and allowed to attach for 24 h on 1% gelatine (Sigma) coated on 96-well plates in complete growth medium under standard conditions (5% CO 2 , 95% humidity, 37 °C). Then, the cells were exposed to Pf TyrRS at the concentrations indicated along with mutant Pf TyrRS or HUVEC alone. The exposure time was 24 hours. Afterwards, the cell culture medium was withdrawn and in each well 10 μl MTT [3-(4,5-dimethylthiazol-2-yl)-2,5-diphenyl tetrazolium bromide, Sigma] stock solution (5 mg ml −1 ) was added, followed by an incubation period of 4 h. Afterwards, 100 μl per well stop solution (40 g SDS per 200 ml 50% DMF (NN-Dimethyformide, Sigma)) was added, followed by an incubation step overnight (37 °C). MTT metabolization as parameter for metabolic activity was recorded spectrophotometrically by Varioskan at 570 nm. Statistical analyses Data are derived from multiple independent experiments done in triplicates. Statistical analyses were conducted using SPSS software and values are presented as mean±s.d. Significant differences between groups were determined by ANOVA followed by Tukey's multiple comparison test (SPSS software). A value of P <0.05 was accepted as an indication of statistical significance. Acccession codes : Coordinates and structure factors for Pf TyrRS have been deposited in the RCSB Protein Data Bank under accession code 3vgj . How to cite this article: Bhatt, T. K. et al . Malaria parasite tyrosyl-tRNA synthetase secretion triggers pro-inflammatory responses. Nat. Commun. 2:530 doi: 10.1038/1522 (2011)